Laminin E8 fragments support efficient adhesion and expansion of dissociated human pluripotent stem cells Human embryonic stem cells (hESCs) and induced pluripotent stem cells (hiPSCs) have the potential to provide an infinite source of tissues for regenerative medicine. Although defined xeno-free media have been developed, culture conditions for reliable propagation of hESCs still require considerable improvement. Here we show that recombinant E8 fragments of laminin isoforms (LM-E8s), which are the minimum fragments conferring integrin-binding activity, promote greater adhesion of hESCs and hiPSCs than do Matrigel and intact laminin isoforms. Furthermore, LM-E8s sustain long-term self-renewal of hESCs and hiPSCs in defined xeno-free media with dissociated cell passaging. We successfully maintained three hESC and two hiPSC lines on LM-E8s in three defined media for 10 passages. hESCs maintained high level expression of pluripotency markers, had a normal karyotype after 30 passages and could differentiate into all three germ layers. This culture system allows robust proliferation of hESCs and hiPSCs for therapeutic applications. Human embryonic stem cells (hESCs) and induced pluripotent stem cells (hiPSCs) have great potential for a wide range of applications in regenerative medicine, and as tools for human disease modelling and drug discovery. However, defined xeno-free and feeder-free systems have not been fully established for the realization of these applications. Several types of defined medium have been developed, which consist of known components and avoid the use of animal products [1] , [2] , [3] , [4] , [5] . However, the widespread use of Matrigel as a culture substrate is potentially problematic [6] . Matrigel is not an optimal substrate because it is derived from mouse Engelbreth–Holm–Swarm tumours and contains many unknown components. Additionally, hESCs usually propagate as colonies in culture, and their passaging involves either enzymatic dissociation by gently pipetting or manual microdissection of the cells [7] . hESC colonies grow as a monolayer and sustain an undifferentiated state, whereas the formation of large aggregates during passaging accelerates their spontaneous differentiation. Thus, it is somewhat difficult to precisely control appropriate dissociation of hESCs while passaging. As a result, conventional colony-based protocols often have considerable variations in culture outcomes. One method to overcome such difficulties might be complete dissociation of hESCs by an optimized and standardized protocol. However, complete dissociation of hESC clumps into single cells causes extensive cell death, and the survival is generally <1% (refs 8 , 9 ). Furthermore, complete cell dissociation is thought to be associated with an increased risk of karyotypic abnormalities [10] , [11] . In this study, we aimed to identify an optimal substrate with the greatest adhesive property for the culture of completely dissociated hESCs and hiPSCs, and we further examined whether it could promote robust propagation of these cells while retaining a normal karyotype. Although there are reports of the replacement of Matrigel with defined substrates, such as small peptides, to allow sustained hESC self-renewal in defined or xeno-free media [3] , [4] , [5] , [12] , [13] , [14] , [15] , [16] , [17] , [18] , considerable improvements and refinements of these substrates are still needed. Laminin, the main component of Matrigel, is a heterotrimeric glycoprotein composed of three covalently linked chains that are termed α, β and γ [19] .Thus far, 15 laminin isoforms formed by various combinations of each chain (α1–α5, β1–β3 and γ1–γ3) have been identified. We have previously shown that human recombinant laminin isoforms (laminin-511, -332 and -111) support hESC proliferation in an undifferentiated state, although laminin-111 shows weak cell adhesive properties [20] . Laminin-511, the first and only alternative substrate with a greater adhesive property for hESCs than that provided by Matrigel, also permits sustained self-renewal of hESCs in xeno-free culture conditions [12] . Typically, procedures for the isolation of native pure laminins from tissues are arduous or highly impractical. Recently, some recombinant laminins have been produced using mammalian expression systems [21] , [22] , [23] , [24] , [25] . However, full-length laminins are large heterotrimeric proteins ( Fig. 1a ), and mass production of these recombinant proteins is still very difficult. Therefore, we examined whether recombinant laminin fragments could support adhesion and undifferentiated proliferation of hESCs and hiPSCs. These fragments are obviously smaller molecules and have a much higher yield compared with that of the full-length protein. 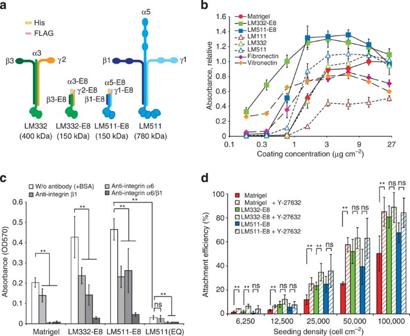Figure 1: Validation of LM-E8s for H9 hESC attachment. (a) Schematic representations of the two LM-E8s and the original intact laminin isoforms. A 6xHis-tag and FLAG-tag were attached to the N-termini of the α and γ chains, respectively, of LM-E8s to facilitate the purification of recombinant LM-E8s. The molecular weights of individual proteins are shown in parentheses. (b) Dose–response adhesion curves of H9 hESCs on various ECMs. LM-E8s at 1.5 μg cm−2showed higher efficiency for supporting the adhesion of dissociated cells than did other matrices. The means of absorbance (OD570) represent the relative number of adherent cells normalized against the values at the maximum effect on Matrigel, which was arbitrarily set as 1. Error bars show the s.e.m. of five independent assays, except for vitronectin, which shows the average of duplicate assays. (c) Inhibition of integrins on LM-E8s. Completely dissociated H9 hESCs were incubated with an integrin-specific blocking antibody for 30 min in mTeSR1 medium. LM511(EQ): an inactive form of LM511-E8. Error bars indicate the s.d. of five individual assays. **P<0.05; ns, non-significant; two-way ANOVA or Tukey’s test. (d) Seeding density-dependent adhesion of H9 hESCs on LM-E8s. LM-E8s showed a higher cell adhesive activity for completely dissociated H9 hESCs than did Matrigel. Completely dissociated cells were incubated on LM-E8s in mTeSR1 medium for 6 h with or without Y-27632. Data represent the means±s.d. of three experiments. **P<0.05; ns, non-significant, two-tailed Student’st-test. Figure 1: Validation of LM-E8s for H9 hESC attachment. ( a ) Schematic representations of the two LM-E8s and the original intact laminin isoforms. A 6xHis-tag and FLAG-tag were attached to the N-termini of the α and γ chains, respectively, of LM-E8s to facilitate the purification of recombinant LM-E8s. The molecular weights of individual proteins are shown in parentheses. ( b ) Dose–response adhesion curves of H9 hESCs on various ECMs. LM-E8s at 1.5 μg cm −2 showed higher efficiency for supporting the adhesion of dissociated cells than did other matrices. The means of absorbance (OD570) represent the relative number of adherent cells normalized against the values at the maximum effect on Matrigel, which was arbitrarily set as 1. Error bars show the s.e.m. of five independent assays, except for vitronectin, which shows the average of duplicate assays. ( c ) Inhibition of integrins on LM-E8s. Completely dissociated H9 hESCs were incubated with an integrin-specific blocking antibody for 30 min in mTeSR1 medium. LM511(EQ): an inactive form of LM511-E8. Error bars indicate the s.d. of five individual assays. ** P <0.05; ns, non-significant; two-way ANOVA or Tukey’s test. ( d ) Seeding density-dependent adhesion of H9 hESCs on LM-E8s. LM-E8s showed a higher cell adhesive activity for completely dissociated H9 hESCs than did Matrigel. Completely dissociated cells were incubated on LM-E8s in mTeSR1 medium for 6 h with or without Y-27632. Data represent the means±s.d. of three experiments. ** P <0.05; ns, non-significant, two-tailed Student’s t -test. Full size image Laminin isoforms bind to multiple receptors on the cell surface, including integrins, syndecans and dystroglycans, of which integrins serve as the major adhesion receptors of hESCs [26] . Laminin-511, -332 and -111 share the characteristic of specific high affinity for α6β1 integrin [27] . Using function-blocking antibodies, α6β1 integrin has been identified as the major cell adhesion receptor for both Matrigel and laminin-511 (refs 12 , 28 ). Furthermore, α6β1 integrin is abundantly expressed by both hESCs [20] and hiPSCs ( Supplementary Fig. S1 ). Thus, we examined whether the integrin-binding site in laminin is solely necessary for the maintenance of hESCs and hiPSCs. Laminin E8 fragments (LM-E8s) are truncated proteins composed of the C-terminal regions of the α, β and γ chains. These truncated proteins contain the active integrin-binding site comprising the laminin globular 1-3 domains of the α chain [21] and the glutamate residue in the C-terminal tail of the γ chain [29] , but lack other activities such as the heparin/heparan sulphate-binding activity, which are associated with intact laminins [21] . Therefore, LM-E8s serve as a functionally minimal form that retains the full capability for binding to α6β1 integrin [30] . When LM-E8s are separated into an α chain and a disulphide-bonded dimer of β and γ chains, they lose their cell adhesive activity [31] , underscoring the requirement for all three chains for their integrin-binding activity. Thus, the integrin-binding site of laminin appears to be a composite epitope composed of multiple polypeptides [32] , thereby making it difficult to recapitulate the integrin-binding site with synthetic peptides modelled on individual laminin subunits. In this study, we produced two recombinant LM-E8s, LM511-E8 from laminin-511 and LM332-E8 from laminin-332, both of which have high cell adhesive properties ( Fig. 1a ), and examined their capabilities as adhesion substrates for hESCs and hiPSCs. Both fragments display stronger adhesion affinities for hESCs and hiPSCs than those of other substrates. Furthermore, LM-E8s enable robust propagation of hESCs and hiPSCs in an undifferentiated state in cultures with defined and xeno-free media using dissociated cell passaging. LM-E8s maximize hESC and hiPSC adhesion Extracellular matrix (ECM) proteins vary considerably in their affinities for receptors, and in protein size and charge. Consequently, different proteins vary in their optimal use as a cell culture support matrix. To determine whether LM511-E8 and LM332-E8 were suitable for hESC and hiPSC adhesion, we first compared the adhesive properties of completely dissociated H9 hESCs and iPS(IMR90)-1 cells in mTeSR1 medium on matrices containing LM511-E8 or LM332-E8 with those on other matrices. Cell adhesion on all matrices showed dose-dependent increases, but with different maxima: 15 μg cm −2 for Matrigel; 3–6 μg cm −2 for intact laminin-511 and -332; and 1.5 μg cm −2 for LM511-E8 and LM332-E8 ( Fig. 1b and Supplementary Figs S2a and S3a ). In agreement with a previous report [12] , adhesion to intact laminin-511 or -332 was higher than that to Matrigel. However, we found that LM511-E8 and LM332-E8 had significantly higher adhesive properties than those of intact laminin-511 and -332. We therefore used LM511-E8 and LM332-E8 at a coating concentration of 1.5 μg cm −2 in subsequent experiments. To confirm that LM511-E8 and LM332-E8 were recognized by α6β1 integrin on the cell surface, we used integrin function-blocking antibodies to investigate whether α6 and/or β1 integrins were required for the adhesion of H9 hESCs to LM-E8-coated substrata in mTeSR1 medium ( Fig. 1c ; Statistical results of multiple comparisons are shown in Supplementary Tables S1a and S1b ). Cell attachment to both LM-E8s was significantly reduced by the addition of antibodies against α6 and/or β1 integrins. We further confirmed that an inactive form of LM511-E8 (LM511(EQ)), in which the glutamic acid residue (E) at the third position from the C-terminus in the γ chain was replaced by a glutamine residue (Q) [29] , showed dramatic abrogation of cell adhesion ( Fig. 1c ). Taken together, these data showed that α6β1 integrin mediated the adhesion of completely dissociated hESCs to LM511-E8 and LM332-E8. Both LM332-E8 and LM511-E8 showed higher adhesion for completely dissociated hESCs or hiPSCs than did Matrigel at various cell densities ( Fig. 1d and Supplementary Fig. S3b ). Furthermore, using the optimal cell density (more than 50,000 cells per cm 2 ), we observed attachment of 40–70% of cells to LM-E8s, which raised the possibility of passaging cultures by completely dissociating hESCs and hiPSCs. It has been previously shown that the Rho-associated protein kinase (ROCK) inhibitor Y-27632 increases the adhesion of dissociated hESCs [33] . However, the effect of Y-27632 on hESC and hiPSC cultures in LM-E8-coated plates was unclear ( Fig. 1d and Supplementary Fig. S3b ). Y-27632 pretreatment before complete dissociation did not significantly improve the attachment of dissociated H9 hESCs on LM-E8s ( Supplementary Fig. S2b ). We therefore concluded that the addition of Y-27632 to the medium was unnecessary for cultures using LM-E8s, unlike attachment onto Matrigel, fibronectin, vitronectin and Synthemax that has a synthetic culture surface consisting of short peptides derived from vitronectin ( Supplementary Fig. S2c ). To focus on the effectiveness of LM-E8s, we did not use Y-27632 in subsequent experiments. In addition, we selected 50,000 cells per cm 2 as the seeding density for passaging hESCs and hiPSCs. LM-E8s support vigorous proliferation in defined media We next examined whether LM-E8s supported undifferentiated growth of completely dissociated hESCs and hiPSCs in mTeSR1 medium. H9 hESC colonies dissociated by a conventional method showed superior attachment to LM-E8s ( Fig. 2a ). Likewise, completely dissociated H9 hESCs showed strong adherence on LM-E8s. Cells quickly adhered and spread on LM-E8-coated substrates, with extending lamellipodium-like protrusions ( Fig. 2b and Supplementary Movies 1 and 2 ). H9 hESCs adhered to LM-E8s promptly recovered cell–cell contacts, formed highly dense colonies ( Fig. 2c ), and showed steady proliferation similar to that of conventional colony cultures ( Fig. 2d ). Similarly, completely dissociated iPS(IMR90)-1 cells also exhibited steady proliferation on LM-E8 fragments ( Supplementary Fig. S3c ). In contrast, completely dissociated H9 hESCs displayed weak adhesion on Matrigel or considerably poor adhesion on fibronectin and vitronectin, although H9 hESC colonies normally adhere to these substrates ( Fig. 2a ). Most dissociated cells on Matrigel, fibronectin and vitronectin remained as single cells and rapidly underwent cell death ( Fig. 2b and Supplementary Movies 3–5 ). In agreement with the cell adhesion and survivability on LM-E8s, molecular analysis revealed that LM-E8s stimulated the signalling pathways downstream of integrins in hESCs and iPSCs. AKT, FAK and ERK1/2, signalling molecules closely associated with cell survival and migration [34] , were activated to a greater extent in cells cultured on LM-E8s than in cells cultured on fibronectin or vitronectin ( Fig. 2e ). Y-27632 treatment abrogated MLC2 phosphorylation regardless of culture substrates, indicating that the signalling pathways promoting cell survival on LM-E8s were not the same as those targeted by Y-27632. Once H9 hESCs adhered on each culture substrate, the cells similarly proliferated at an invariable rate that was regardless of the culture substrate, cluster size and Y-27632 treatment ( Fig. 2d and Supplementary Fig. S2d ). Therefore, the expansion efficiency was simply dependent on the initial adhesion efficiency and passaging ratio. LM-E8s allowed a higher passaging ratio during subculture, which was approximately 1:10 compared with 1:4 for conventional colony culture. Indeed, LM-E8s yielded more than 200-fold of the number of cells compared with that obtained by conventional culture over a 1-month period ( Fig. 2f ). Thus, LM-E8s enabled rapid expansion of completely dissociated hESCs and hiPSCs by supporting robust adhesion and rapid cell expansion. 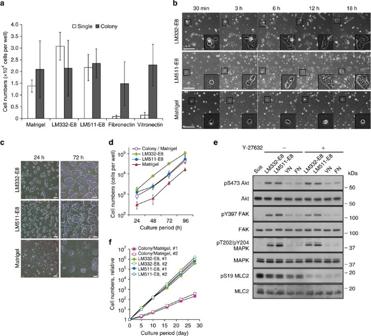Figure 2: LM-E8s support undifferentiated proliferation in defined medium. (a) Distinct cell survival of H9 hESCs depending on ECMs. Data represent the numbers of live cells at 24 h after seeding 3.75 × 104cells as single cells (single) or colonies (colony). (b) Serial phase-contrast images of H9 hESCs on LM-E8s or Matrigel in mTeSR1 medium at initial attachment. Images at the bottom right show an enlarged view of enclosed boxes. Note that dissociated H9 hESCs promptly extended and reached neighbouring cells on LM-E8s, but failed cellular extension on Matrigel. See alsoSupplementary Movies 1–5. (c) Phase-contrast images of H9 hESCs in mTeSR1 medium on LM-E8s or Matrigel during the growth phase. (d) Short-term growth curves of H9 hESCs on LM-E8s in mTeSR1 medium. Dissociated H9 hESCs on LM-E8s proliferated and had a similar growth rate as that in conventional colony culture during logarithmic growth. Data represent the means±s.d. of three individual experiments. (e) Detection of phosphorylated proteins associated with cell adhesion by western blot analysis. Cell lysates were prepared from H9 hESCs incubated for 1 h on each substrate with or without Y-27632. Sus, dissociated H9 hESCs incubated for 1 h in suspension; FN, fibronectin; VN, vitronectin. (f) Long-term growth curves of H9 hESCs on LM-E8s in mTeSR1 medium. The numbers of seeded cells at the initial passage were converted to 1, and the counted cell numbers at each passage are shown as cumulative cell numbers. Note that dissociation culture on LM-E8s resulted in a more than 200-fold increase in cell numbers relative to conventional colony culture over 1 month. Scale bars, 200 μm. Figure 2: LM-E8s support undifferentiated proliferation in defined medium. ( a ) Distinct cell survival of H9 hESCs depending on ECMs. Data represent the numbers of live cells at 24 h after seeding 3.75 × 10 4 cells as single cells (single) or colonies (colony). ( b ) Serial phase-contrast images of H9 hESCs on LM-E8s or Matrigel in mTeSR1 medium at initial attachment. Images at the bottom right show an enlarged view of enclosed boxes. Note that dissociated H9 hESCs promptly extended and reached neighbouring cells on LM-E8s, but failed cellular extension on Matrigel. See also Supplementary Movies 1–5 . ( c ) Phase-contrast images of H9 hESCs in mTeSR1 medium on LM-E8s or Matrigel during the growth phase. ( d ) Short-term growth curves of H9 hESCs on LM-E8s in mTeSR1 medium. Dissociated H9 hESCs on LM-E8s proliferated and had a similar growth rate as that in conventional colony culture during logarithmic growth. Data represent the means±s.d. of three individual experiments. ( e ) Detection of phosphorylated proteins associated with cell adhesion by western blot analysis. Cell lysates were prepared from H9 hESCs incubated for 1 h on each substrate with or without Y-27632. Sus, dissociated H9 hESCs incubated for 1 h in suspension; FN, fibronectin; VN, vitronectin. ( f ) Long-term growth curves of H9 hESCs on LM-E8s in mTeSR1 medium. The numbers of seeded cells at the initial passage were converted to 1, and the counted cell numbers at each passage are shown as cumulative cell numbers. Note that dissociation culture on LM-E8s resulted in a more than 200-fold increase in cell numbers relative to conventional colony culture over 1 month. Scale bars, 200 μm. Full size image Using our culture protocol with LM-E8s and two chemically defined media (mTeSR1 and StemPro), three hESC lines (H9, HES3 and KhES-1) and two hiPSC lines (iPS(IMR90)-1 and 253G1) showed robust proliferation for at least 10 serial passages. Flow cytometric analysis further indicated that the majority of dissociated hESCs and hiPSCs cultured on LM-E8s expressed pluripotency markers SSEA-3, SSEA-4, Tra-1-60, Tra-1-81, GCTM2 and Tra-2-54, with only low level of expression of the differentiation marker SSEA-1 ( Fig. 3 ). It has been reported that N2B27 medium is less robust for hESC maintenance, compared with two other media [2] , but almost all hESCs and hiPSCs, except for KhES-1, cultured on LM-E8s showed undifferentiated growth in N2B27 medium. We karyotyped 50 randomly selected cells after G-banding of each cell line for all experiments at passage 10. Cells propagated on LM-E8s after complete dissociation had normal karyotypes ( Table 1 and Supplementary Fig. S4a, b ). Using multiplex fluorescence in situ hybridization (M-FISH) analysis, we showed that completely dissociated H9 hESCs and iPS(IMR90)-1 cells had a normal karyotype after 30 and 20 passages on LM-E8s, respectively ( Supplementary Fig. S4c–f ). 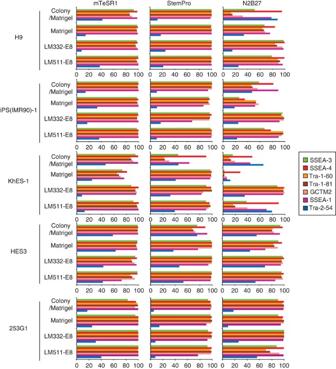Figure 3: Flow cytometric analysis of hESC or hiPSC lines. Three hESC lines (H9, HES3 and KhES-1) and two hiPSC line (iPS(IMR90)-1 and 253G1) were cultured on LM-E8s after complete dissociation. These cells maintained higher expression levels of the undifferentiated markers, compared with that on Matrigel with either colony or complete dissociation culture. Undifferentiated markers: SSEA-3, SSEA-4, Tra-1-60, Tra-1-81, GCTM2 and Tra-2-54. Differentiation marker: SSEA-1. Data were collected from cells cultured for 10 passages. The percentages of positive cells are indicated on the graph. Figure 3: Flow cytometric analysis of hESC or hiPSC lines. Three hESC lines (H9, HES3 and KhES-1) and two hiPSC line (iPS(IMR90)-1 and 253G1) were cultured on LM-E8s after complete dissociation. These cells maintained higher expression levels of the undifferentiated markers, compared with that on Matrigel with either colony or complete dissociation culture. Undifferentiated markers: SSEA-3, SSEA-4, Tra-1-60, Tra-1-81, GCTM2 and Tra-2-54. Differentiation marker: SSEA-1. Data were collected from cells cultured for 10 passages. The percentages of positive cells are indicated on the graph. Full size image Table 1 Summary of karyotypic analysis. Full size table To assess the pluripotency of hESCs that had been cultured on LM-E8s in mTeSR1 medium for 10 passages, the cells were treated with the growth factors described in the Methods . We found that hESCs could differentiate into ectoderm (βIII tubulin), mesoderm (α-smooth muscle actin) or endoderm (α-fetoprotein), as determined by immunohistochemical analyses ( Fig. 4a ). Furthermore, reverse transcriptase PCR (RT–PCR) analysis showed that, when hESCs were placed in suspension culture, they formed embryoid bodies with increased expression of gene markers for all three germ layer lineages after 10 days of incubation ( Fig. 4b ). Similar results were obtained for iPS(IMR90)-1 cells cultured on LM-E8s ( Supplementary Fig. S5 ). We further confirmed that hESCs cultured on LM-E8s in mTeSR1 medium for 25 passages formed teratomas consisting of all three germ layers, including neuroepithelium (ectoderm), intestinal epithelium (endoderm) and cartilage (mesoderm) ( Fig. 4c ). 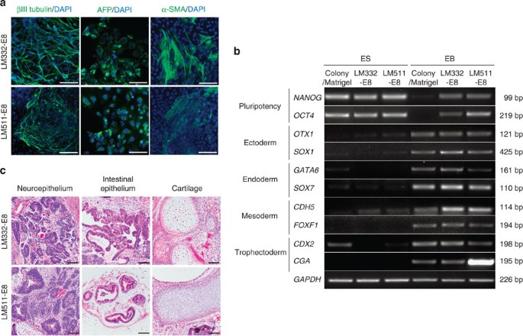Figure 4: LM-E8s sustain pluripotency in defined medium. (a) Immunostaining for markers of the three germ layers in differentiating H9 hESCs cultured on LM-E8s in mTeSR1 medium after 10 passages: ectoderm (βIII tubulin), endoderm (alpha-fetoprotein (AFP)), and mesoderm (α-smooth muscle actin (SMA)). (b) RT–PCR analysis of marker genes for the differentiation of embryoid bodies. H9 hESCs were cultured in mTeSR1 medium for 10 passages on LM-E8s after complete dissociation, or on Matrigel after colony dissociation. Cells were then allowed to form embryoid bodies for 10 days. (c) Teratomas consisting of the three germ layers developed following the transfer of H9 hESCs cultured on LM-E8s after 25 passages in mTeSR1 medium. Cells were injected into the testes of SCID mice. After 8 weeks, the fate of the cells was analysed. Haematoxylin and eosin staining showed differentiation into various tissues including neuroepithelium (ectoderm), intestinal epithelium (endoderm) and cartilage (mesoderm). Scale bars, 200 μm. Figure 4: LM-E8s sustain pluripotency in defined medium. ( a ) Immunostaining for markers of the three germ layers in differentiating H9 hESCs cultured on LM-E8s in mTeSR1 medium after 10 passages: ectoderm (βIII tubulin), endoderm (alpha-fetoprotein (AFP)), and mesoderm (α-smooth muscle actin (SMA)). ( b ) RT–PCR analysis of marker genes for the differentiation of embryoid bodies. H9 hESCs were cultured in mTeSR1 medium for 10 passages on LM-E8s after complete dissociation, or on Matrigel after colony dissociation. Cells were then allowed to form embryoid bodies for 10 days. ( c ) Teratomas consisting of the three germ layers developed following the transfer of H9 hESCs cultured on LM-E8s after 25 passages in mTeSR1 medium. Cells were injected into the testes of SCID mice. After 8 weeks, the fate of the cells was analysed. Haematoxylin and eosin staining showed differentiation into various tissues including neuroepithelium (ectoderm), intestinal epithelium (endoderm) and cartilage (mesoderm). Scale bars, 200 μm. Full size image Thus, our new culture method using completely dissociated cells on LM-E8s supported long-term maintenance and efficient cell expansion of hESCs and hiPSCs in an undifferentiated state. LM-E8s support vigorous proliferation in xeno-free medium The final goal of this study was to characterize LM-E8s as substrates that support hESCs in a sustainable undifferentiated state under a xeno-free culture condition. We cultured completely dissociated H9 hESCs and 253G1 iPSCs on LM511-E8 or LM332-E8 in TeSR2 medium that is chemically defined and animal protein free. Dissociated H9 hESCs tightly adhered on LM-E8s in TeSR2 medium ( Fig. 5a ). Similarly to the results described for defined media, we found that H9 hESCs and 253G1 iPSCs proliferated robustly for more than 30 and 10 passages, respectively. Flow cytometric analysis also confirmed that the cells retained their undifferentiated state ( Fig. 5b and Supplementary Fig. S6a ). RT–PCR analysis of H9 hESCs and 253G1 iPSCs cultured on LM-E8s after complete dissociation showed that the expression of pluripotency markers, including NANOG and OCT4 , remained high, whereas the expression of differentiation lineage markers was suppressed ( Fig. 5c and Supplementary Fig. S6b ). H9 hESCs and 253G1 iPSCs had a normal karyotype after 35 and 10 serial passages, as indicated by G-band analysis ( Supplementary Fig. S7a–d ), and M-FISH analysis corroborated these findings ( Supplementary Fig. S7e,f ). In addition, we confirmed the pluripotency of hESCs cultured on LM-E8s by their ability to form teratomas comprising all three germ layers ( Fig. 5d ). 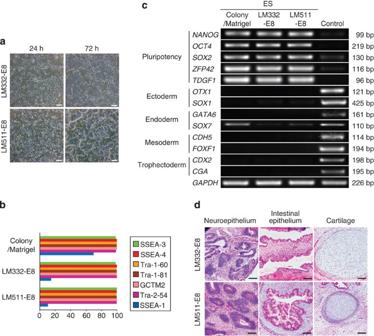Figure 5: LM-E8s sustain the pluripotency in xeno-free TeSR2 medium. (a) Phase-contrast images of H9 hESCs. Dissociated H9 hESCs in TeSR2 medium reformed clusters (24 h) and actively proliferated (72 h). (b) Flow cytometric profiles of H9 hESCs cultured on LM-E8s for 34 passages after complete dissociation, or on Matrigel for 30 passages after colony dissociation. H9 hESCs maintained expression of markers of the undifferentiated state. Numbers indicate percentages of cells that were positive for surface markers. (c) RT–PCR analysis of the expression of pluripotency marker genes in H9 hESCs cultured in TeSR2 medium. H9 hESCs cultured for 30 passages on LM-E8s after complete dissociation maintained high-level expression of pluripotency marker genes, while differentiation lineage marker genes were suppressed. Embryoid bodies derived from H9 hESCs cultured as colonies in mTeSR1 medium were used as the control to assess differentiation. (d) Teratomas consisting of the three germ layers developed from H9 hESCs cultured on LM-E8s for 34 passages in TeSR2 medium after complete dissociation. Cells were injected into the testes of SCID mice. After 8 weeks, the fate of the cells was analysed. Haematoxylin and eosin staining showed differentiation into various tissues including neuroepithelium (ectoderm), intestinal epithelium (endoderm) and cartilage (mesoderm). Scale bars, 200 μm. Figure 5: LM-E8s sustain the pluripotency in xeno-free TeSR2 medium. ( a ) Phase-contrast images of H9 hESCs. Dissociated H9 hESCs in TeSR2 medium reformed clusters (24 h) and actively proliferated (72 h). ( b ) Flow cytometric profiles of H9 hESCs cultured on LM-E8s for 34 passages after complete dissociation, or on Matrigel for 30 passages after colony dissociation. H9 hESCs maintained expression of markers of the undifferentiated state. Numbers indicate percentages of cells that were positive for surface markers. ( c ) RT–PCR analysis of the expression of pluripotency marker genes in H9 hESCs cultured in TeSR2 medium. H9 hESCs cultured for 30 passages on LM-E8s after complete dissociation maintained high-level expression of pluripotency marker genes, while differentiation lineage marker genes were suppressed. Embryoid bodies derived from H9 hESCs cultured as colonies in mTeSR1 medium were used as the control to assess differentiation. ( d ) Teratomas consisting of the three germ layers developed from H9 hESCs cultured on LM-E8s for 34 passages in TeSR2 medium after complete dissociation. Cells were injected into the testes of SCID mice. After 8 weeks, the fate of the cells was analysed. Haematoxylin and eosin staining showed differentiation into various tissues including neuroepithelium (ectoderm), intestinal epithelium (endoderm) and cartilage (mesoderm). Scale bars, 200 μm. Full size image Stem cell–ECM interactions are important for maintaining stem cell adhesion, survival and self-renewal both in vivo and in vitro . The development of an ECM that sustains hESC and hiPSC cultures still requires substantial effort, particularly to avoid the use of feeder cells. In this study, we have demonstrated that LM-E8s support stronger adhesion of hESCs and hiPSCs than do other substrates, including Matrigel and intact laminin-511. We showed that LM-E8s enabled rapid and steady expansion of these cells. Furthermore, the cells cultured on LM-E8s for more than 30 passages in defined xeno-free media maintained an undifferentiated state and retained a normal karyotype and pluripotency. The adhesion of these cells to LM-E8s is primarily α6β1 integrin-dependent, because a function-blocking antibody against α6β1 integrin strongly inhibits the cell adhesion. Furthermore, LM511(EQ), a mutant LM-E8 that cannot bind to α6β1 integrin owing to a single amino-acid substitution [29] , does not support the adhesion of hESCs. Thus, we believe that the interaction of LM-E8s with α6β1 integrin is the principal route for binding to hESCs and promotion of proliferation in an undifferentiated state. Although laminin-511 was shown to be a potential substrate for feeder-free culture of hESCs, intact laminin-511 is a large heterotrimeric protein of 780 kDa ( Fig. 1a ) and requires three independent transfections of expression vectors encoding the α, β and γ chains, each of which is larger than 10 kb, for recombinant protein production. It is therefore an arduous protocol to produce recombinant laminin-511 in sufficient quantities for the clinical application of hESCs. Here, we have shown that LM-E8s, the minimum structure harbouring the full integrin-binding activity of laminins, are superb substrates for the long-term culture of hESCs, with a substantial advantage over intact laminin-511 and laminin-332. LM-E8s are much smaller and easier to produce recombinantly than intact laminins. Indeed, the smaller size of LM-E8s significantly improves recombinant protein expression, allowing LM-E8s to yield more than five times more recombinant protein than intact laminin-511 (see Methods ). In addition, LM-E8s can be easily purified using 6xHis- and FLAG-tags attached to the α and γ chains, respectively ( Fig. 1a ). This method reduces the time required for purification and increases the purity of recombinant proteins, compared with intact laminin-511. These advantages endow LM-E8s with a greater potential for scaled-up production, compared with intact laminins. Importantly, LM-E8s have a higher adhesion affinity for hESCs than do intact laminin-511 and laminin-332, although the reasons for this property are yet to be fully determined. The smaller size of LM-E8s may allow them to pack more closely to each other on the substrate and thereby increases the adhesiveness of the substrate for hESC attachment by either increasing the ligand-binding affinity of integrins and/or enhancing the signalling events triggered by integrin clustering. Several groups have reported that vitronectin and one of its variants (VTN-NC) supports the maintenance of hESCs via αVβ5 integrin [4] , [13] . The binding affinity of vitronectin to αVβ5 integrin was 10-fold lower than that of LM-E8 to α6β1 integrin (Yuya Sato, K.S., unpublished data), suggesting that vitronectin is potentially inferior for hESC adhesion compared with LM-E8s. Indeed, although hESCs and hiPSCs have been cultured as colonies on fibronectin and vitronectin [1] , [13] , [35] , [36] , hESCs and hiPSCs that had been completely dissociated showed less adhesion ( Fig. 2a ). It has been reported that AKT, ERK1/2 and kinases interacting with FAK are highly phosphorylated in human pluripotent stem cells [37] . Furthermore, it is well known that AKT and FAK, stimulated via integrin activation, perform numerous cell survival functions [34] . The phosphorylation of AKT, FAK and ERK1/2 confirms that LM-E8s have the potential to promote the survival of completely dissociated hESCs by robust adhesion via integrins, whereas vitronectin and fibronectin are unfavourable for culturing of completely dissociated hESCs and hiPSCs. The ROCK inhibitor Y-27632 has been shown to increase the survival of dissociated hESCs [33] . Tsutsui et al. . [5] reported maintenance of hESCs on a fibronectin-coated surface by dissociated cell passaging, but their method requires a high dose of Y-27632 for cell attachment to fibronectin. It should be noted that a high concentration of Y-27632 increases toxicity and leads to a reduction of hESC numbers in some cases [38] . Additionally, the maintenance of hESCs on fibronectin requires constant administration of Y-27632, even after cell attachment. In contrast, our method using LM-E8s does not require Y-27632 administration owing to sufficient stimulation of cell survival from the culture substrate. This method might be advantageous not only for supporting cell expansion but also for use in drug screening studies. This is because LM-E8s not only improve the culture condition to avoid transient adverse effects of untargeted chemicals, such as Y-27632, but also allow uniform seeding of routine numbers of hESCs and hiPSCs. Therefore, LM-E8s are an appropriate culture substrate for the culture of completely dissociated hESCs and hiPSCs. Although LM-E8s ensured hESC survival just after cell seeding, single hESCs exhibited poor survival over prolonged time periods, even on LM-E8s. It is known that E-cadherin signalling, which arises from cell–cell contact, has a key role in the self-renewal of hESCs as well as the generation of hiPSCs [39] , [40] , [41] . LM-E8 signalling may be insufficient for prolonged survival of single hESCs, but LM-E8s enabled hESCs to actively migrate, and the cells aggregated promptly and restored cell–cell contacts to form small colonies within 24 h of culture initiation ( Figs 2b, c and ). FAK is known to perform multiple functions and regulates cell migration [42] . The increased phosphorylation of FAK is indicative of active migration of dissociated hESCs on LM-E8s. It has been recently reported that cell–cell contact promotes hESC survival, and Y-27632 treatment accelerates the migration of hESCs to reconstruct cell–cell contacts [43] . Here, we show that LM-E8s also activated dissociated hESC migration, but the mechanism is different from that of Y-27632 treatment, as shown by the MLC2 phosphorylation analysis. Collectively, LM-E8s support not only strong adhesion to hESCs and hiPSCs but also promote cell–cell contact by inducing their migration ability, thereby ensuring cell survive and proliferation. Thus, our new protocol improves the adhesion of hESCs and hiPSCs and allows efficient propagation in a simple and rapid manner. In conclusion, we demonstrate a defined xeno- and feeder-free culture system for hESCs and hiPSCs. LM-E8s derived from laminin isoforms support increased adhesion, survival, self-renewal and differentiation of hESCs. This simple culture system should facilitate bulk proliferation of hESCs and hiPSCs under defined xeno-free conditions. We believe that our protocol will be useful for clinical applications of hESCs and hiPSCs in compliance with good manufacturing practice and/or current good tissue practice. Preparation of ECMs Recombinant human laminins, laminin-111, -332 and -511 and LM-E8s (LM322-E8 and LM511-E8) were produced using a FreeStyle 293 Expression System (Invitrogen) as described previously [21] , [29] , [30] . Laminin-111, -332 and -511 and LM-E8s were filtered through 0.22-μm-pore-sized Ultrafree-CL Centrifugal Filter Units (Millipore) for sterilization. Using these methods, we purified an average of 0.74 mg intact LM511 ( n =5) and 4.1 mg LM511-E8 ( n =4) from 1 l of culture supernatant. Thus, the yield was much higher for LM511-E8 (5.5-fold in terms of weight, or 27.7-fold per mol) than for intact laminin. Furthermore, purification of intact laminin-511 required 1–2 weeks, whereas purification of LM-E8s required only 2–3 days. Human fibronectin and vitronectin were purified from plasma, as described elsewhere [44] , [45] . Matrigel (Growth Factor Reduced) was purchased from BD Biosciences. Coating of matrices For the dose–response binding assay, 96-well flat-bottomed plates (non-treated, BD Falcon) were precoated with each of the matrices at a concentration of 0–25 μg cm −2 for 3 h at room temperature just before cell seeding. For other experiments, we used 48-well plates (non-treated, BD Falcon) precoated with LM-E8s, fibronectin, or vitronectin at 1.5 μg cm −2 or Matrigel at 25 μg cm −2 for 3 h at room temperature for the culture of hESCs and hiPSCs. For conventional colony passaging as an experimental control, 12-well plates were coated with Matrigel at 25 μg cm −2 . Coated dishes were not rinsed with buffer before use. To dilute the ECMs, Dulbecco’s PBS was used for laminin-111, -332 and -511, LM-E8s, fibronectin and vitronectin. DMEM/F12 was used to dilute Matrigel. Preparation of defined media Commercially available defined media, mTeSR1 (mTeSR1; Stem Cell Technologies) and StemPro hESC SFM (StemPro, Invitrogen) and xeno-free medium, TeSR2 (TeSR2; Stem Cell Technologies), were used according to the manufacturer’s instructions and freshly prepared every day. N2B27 medium was prepared daily, according to previous reports [1] , [2] , and was composed of DMEM/F12 (Sigma, D6421), 1 × N2 supplement (Invitrogen), 1 × B27 supplement (Invitrogen), 1 mM non-essential amino acids (Sigma, M7145), 1 mM L -glutamine (Sigma, G7513), 0.1 mM 2-mercaptoethanol (Invitrogen) and 100 ng ml −1 FGF-2 (Wako, Japan, 060-04543). Cell culture hESC lines, KhES-1 at passage 22 and HES3 at passage 100, and hiPSC line 253G1 at passage 50 were maintained as previously described on mitomycin-C-treated mouse embryonic fibroblast (MEF) feeder cells [46] . The hESC line H9 (WA09) at passage 36, hiPSC line iPS (IMR90) clone 1 (iPS(IMR90)-1) at passage 80 and iPS (foreskin) line at passage 64 were purchased from the National Stem Cell Bank. Cells were maintained in accordance with National Stem Cell Bank protocols, except for the use of mitomycin-C-treated MEFs from the ICR strain at a density of 3.2 × 10 4 cells per cm 2 . Experimental control cells were obtained from conventional colony cultures that were maintained as follows. Near-confluent cells were incubated with 2 mg ml −1 dispase in DMEM/F12 at 37 °C for 2 min, and then rinsed twice with DMEM/F12. After addition of defined medium, weakly adherent colonies were detached using a cell scraper. Cells were collected and centrifuged at 200 g for 3 min at 4 °C. Small colonies were then passaged into Matrigel-coated vessels at a ratio of 1:4. Colonies showing morphological differentiation were manually removed under a microscope during each passage, except at the time of analysis. Completely dissociated cells were cultured after preculture in the appropriate defined medium for one passage on Matrigel-coated dishes to remove MEF feeders. This stage was defined as passage 0. Near-confluent cell clusters were treated with 4.8 mM EDTA/PBS for 2–5 min at room temperature and then TrypLE Select (Invitrogen) for 1 min at 37 °C. Cells in defined medium were pipetted to disperse the cells completely. After centrifugation at 200 g for 3 min at 4 °C, cells were seeded at the appropriate density (5 × 10 4 cells per cm 2 for passaging or as indicated) into new culture vessels precoated with each matrix. The medium was changed daily for all experiments. hESCs and hiPSCs on LM-E8s were subcultured every 4–6 days, and those on Matrigel every 6–8 days. Time-lapse recording For time-lapse recording during initial attachment, completely dissociated H9 hESCs were seeded onto LM-E8-, fibronectin-, vitronectin- or Matrigel-coated 35-mm dishes at 2.5 × 10 4 cells per cm 2 in mTeSR1 medium. Recording began at 5 min after cell seeding and continued for 24 h. Movies were edited using AxioVisio software. Cell adhesion assay Dose–response binding assays were performed using a protocol described elsewhere [13] , with some modification. Briefly, hESCs or hiPSCs were cultured for one passage on Matrigel in mTeSR1 medium to remove feeder cells, and then the cells were detached using TrypLE Select, collected and counted. A total of 5 × 10 4 cells were seeded into each well of 96-well plates coated with the matrices described above. After 6 h of incubation, non-adherent cells were removed by rinsing the plates twice with DMEM/F12, and the remaining adherent cells were fixed with 10% formalin for 15 min, and postfixed in 100% ethanol for 5 min at room temperature. Cells were then stained with 0.4% crystal violet in methanol for 5 min at room temperature. After washing extensively with demineralized water, the remaining cells were solubilized by adding 100 μl of 1% SDS, and the optical density at 570 nm was measured by a multiwell plate reader. For the functional inhibition assay of integrins, H9 hESCs were seeded into each well of 96-well plates coated with the various matrices including LM511(EQ) in the presence or absence of 2 μg ml −1 integrin-blocking antibodies, anti-α6 integrin (R&D systems) and/or anti-β1 integrin (R&D systems). After 30 min of incubation, adherent cells were screened as described above for the dose–response assay. For the seeding density assay, hESCs or hiPSCs were precultured in mTeSR1 medium on Matrigel-coated vessels for one passage to remove feeder cells. Cells were detached using an EDTA solution and TrypLE Select as described above. Cells were seeded into 48-well plates coated with LM-E8s or Matrigel. After 6 h of incubation, non-adherent cells were rinsed twice with prewarmed DMEM/F12, and the remaining adherent cells were detached using 0.25% Trypsin/EDTA. Viable cells were counted by trypan blue exclusion. For the proliferation assay, dissociated single cells were seeded at a density of 4 × 10 4 cells per cm 2 , and viable cells were counted every 24 h as described above. In parallel, colonies were seeded on 24-well plates coated with Matrigel at the same cell density. To evaluate Y-27632 pretreatment, H9 hESCs cultured on Matrigel in mTeSR1 medium were incubated with 10 μM Y-27632 (Wako, 253-00513) for 1 h just before cell detachment. Together with the cultures without Y-27632 pretreatment, cells were detached by EDTA and TrypLE Select treatment and then seeded in multiwell plates coated with substrates in mTeSR1 medium containing 10 μM Y-27632. To evaluate the effect of Y-27632 treatment on cell proliferation, H9 hESCs after complete dissociation or as colonies were seeded at a density of 5 × 10 4 cells per cm 2 with or without 10 μM Y-27632 in 48-well plates coated with each substrate. Viable cells were counted every 24 h. To evaluate a derivation of vitronectin, a Synthemax-R Surface 6-well plate (Corning) was used as a substrate. Flow cytometric analysis Cells were dissociated by treatment with 4.8 mM EDTA/PBS for 2–5 min, followed by further treatment with a 0.05% trypsin/EDTA solution for 1 min. After two washes with DMEM/10% FBS and one wash with staining buffer (0.1% BSA/PBS), 1 × 10 5 cells were incubated for 30 min at 4 °C with primary antibodies diluted in staining buffer. Cells were then rinsed twice with staining buffer and incubated for 30 min at 4 °C with secondary antibodies diluted in staining buffer. Then, cells were rinsed twice with staining buffer, and counterstained with propidium iodide just before analysis. Fluorescence intensities were analysed on a FACSCalibur flow cytometer (Becton Dickinson), and the FL-1 positive ratios in the propidium iodide-negative region were monitored using Cell Quest software. The following primary antibodies were used: SSEA-3 (2 μg ml −1 ; Developmental Studies Hybridoma Bank (DSHB), SSEA-4 (1 μg ml −1 ; DSHB), Tra-1-60 (1 μg ml −1 ; Chemicon), Tra-1-81 (1 μg ml −1 ; Chemicon), GCTM2 (1 μg ml −1 ; Chemicon), Tra-2-54 (1 μg ml −1 , DSHB), and SSEA-1 (2 μg ml −1 ; DSHB). Anti-mouse Ig/FITC conjugated (10 μg ml −1 ; Becton Dickinson) and anti-rat IgM/Alexa 488 conjugated (1 μg ml −1 ; Molecular Probes) were used as secondary antibodies. Karyotyping hESCs and hiPSCs were treated with 100 ng ml −1 colcemid (Invitrogen) for 2–3 h. After dissociation in 0.25% trypsin/EDTA solution, cells were treated with a hypotonic solution and then fixed in Carnoy’s solution. Cells were spread onto glass slides and stained with Giemsa. Chromosome spreads were analysed by randomly counting 50 cells using the Ikaros Karyotyping System (META system). M-FISH analysis was performed using the 24XCyte Human Multicolor FISH (mFISH) Probe Kit (META system) following the manufacturer’s instructions, and analysed by ISIS software (META system). Statistical analysis The statistical significance of differences was determined by the two-tailed Student’s t -test for two group comparisons, or two-way analysis of variance (two-way ANOVA) for multiple comparisons followed by Tukey’s test. Differences with a value of P <0.05 were considered significant. Other methods See Supplementary Methods and Supplementary Table S2 for remaining methods, including semi-quantitative RT–PCR, the differentiation assay, immunofluorescence staining and immunoblotting. How to cite this article: Miyazaki, T. et al. . Laminin E8 fragments support efficient adhesion and expansion of dissociated human pluripotent stem cells. Nat. Commun. 3:1236 doi: 10.1038/ncomms2231 (2012).